Alpha kinase 1 controls intestinal inflammation by suppressing the IL-12/Th1 axis 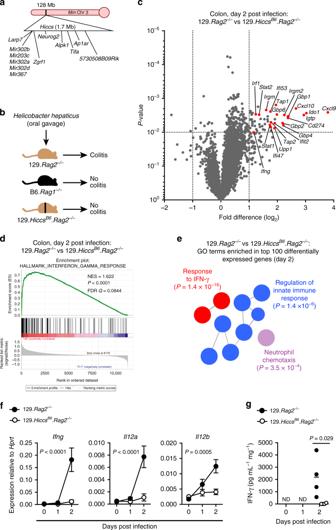Fig. 1 129.Rag2−/−mice rapidly activate interferon-gamma signaling following infection withHh.aSchematic of theHiccslocus, which regulates sensitivity toHh-driven innate colitis.bColitis phenotypes afterHhinfection of B6.Rag1−/−, 129.Rag2−/−, or congenic 129.Rag2−/−mice bearing aHiccslocus that matches the B6 genotype (129.HiccsB6.Rag2−/−).c–eTranscriptomic profiling of whole-colon tissue from 129.Rag2−/−and 129.HiccsB6.Rag2−/−mice 2 days after oralHhinfection (n= 4 per group).cTornado plot displaying log2fold differences in 129.Rag2−/−versus 129.HiccsB6.Rag2−/−mice. IFN-γ-regulated genes are indicated in red.dGene set enrichment analysis (GSEA), showing enrichment of the “interferon-gamma response” hallmark gene set in colon tissue from 129.Rag2−/−mice.eThe top 100 differentially expressed genes (high in 129.Rag2−/−mice) were analyzed for gene ontology (GO) term enrichment using ClueGO. The most highly enriched GO terms are shown, with lead terms and associatedp-values indicated.fRT-qPCR analysis of whole-colon gene expression afterHhinfection. Data analyzed by two-way ANOVA (n= 4 per group per time point).P-values indicate day 2 comparisons corrected with Sidak’s multiple comparisons tests (DF = 17 for each comparison).gIFN-γ secretion by colon explant tissue cultured overnight ex vivo at steady state or followingHhinfection. ND no IFN-γ detected in culture supernatant. Data (Hhday 2) analyzed by Mann–Whitney test (n= 4 per group/timepoint). Data inc–gare from one experiment Inflammatory bowel disease (IBD) are heterogenous disorders of the gastrointestinal tract caused by a spectrum of genetic and environmental factors. In mice, overlapping regions of chromosome 3 have been associated with susceptibility to IBD-like pathology, including a locus called Hiccs . However, the specific gene that controls disease susceptibility remains unknown. Here we identify a Hiccs locus gene, Alpk1 (encoding alpha kinase 1), as a potent regulator of intestinal inflammation. In response to infection with the commensal pathobiont Helicobacter hepaticus ( Hh ), Alpk1-deficient mice display exacerbated interleukin (IL)-12/IL-23 dependent colitis characterized by an enhanced Th1/interferon(IFN)-γ response. Alpk1 controls intestinal immunity via the hematopoietic system and is highly expressed by mononuclear phagocytes. In response to Hh , Alpk1 −/− macrophages produce abnormally high amounts of IL-12, but not IL-23. This study demonstrates that Alpk1 promotes intestinal homoeostasis by regulating the balance of type 1/type 17 immunity following microbial challenge. Inflammatory bowel disease (IBD) pathogenesis is mechanistically complex and includes elements of genetic susceptibility, immune dysregulation, environmental factors, and the microbiome. As with humans, colitis in mice is strongly influenced by host genetics, such that different inbred strains exhibit widely divergent phenotypes in models of IBD [1] , [2] . For example, whereas 129SvEv. Rag2 −/− mice develop aggressive colitis following infection with Hh , C57BL/6 .Rag1 −/− mice do not [3] . 129SvEv mice deficient for the Wiskott-Aldrich syndrome protein ( Was −/− ) are also susceptible to spontaneous colitis [4] . In recent years, two loci on chromosome 3—termed “cytokine-dependent colitis susceptibility locus” ( Cdcs1 ) in C3H/HeJBir mice, and “ Helicobacter hepaticus -induced colitis and associated cancer susceptibility” ( Hiccs ) in 129SvEv mice —have been identified as the critical genetic determinants of colitis susceptibility in these strains [2] , [3] , [5] , [6] , [7] , [8] . The Cdcs1 locus was first identified in the context of interleukin-10 deficient ( Il10 −/− ) mice over 10 years ago [5] , [8] , and also controls spontaneous colitis in C57BL/6 .Tbx21 −/− Rag2 −/− (TRUC) mice [9] . The Hiccs locus, located in a similar region of chromosome 3, controls susceptibility to Hh -induced colitis and eventual onset of colitis-associated colorectal cancer [3] . The ability of the Cdcs1 and Hiccs loci to control colitis susceptibility in several mechanistically distinct models suggests that they include one or more critical immunoregulatory genes. However, individual Cdcs1 / Hiccs -related genes have not been directly studied in the context of intestinal inflammation. A Hiccs locus gene, Alpha kinase 1 ( Alpk1 ), has multiple non-synonymous single nucleotide differences in its coding region between the colitis-susceptible 129SvEv and the resistant C57BL/6 mouse strains [3] . We previously showed that Alpk1 expression is upregulated in response to inflammatory stimuli in myeloid cells [3] . Also, single nucleotide polymorphisms (SNPs) in the human ALPK1 gene have been linked to a variety of inflammatory conditions, including gout and chronic kidney disease [10] , [11] . More recently, in vitro studies suggested that Alpk1 mediates pathogen-induced IL-8 expression in gastric epithelial cells [12] , [13] , making it a relevant gene to explore in the context of gut inflammation. In this study, we further refine the Cdcs1 locus and identify a core colitis-determining region that is essentially identical to the Hiccs locus. To address a potential role for Alpk1 in regulation of intestinal homoeostasis, we have generated Alpk1-deficient mice. We show that Alpk1 deficiency leads to severe colitis and an exaggerated Th1 immune response in mice infected with the intestinal pathobiont Helicobacter hepaticus . We further demonstrate that Alpk1 exerts its anti-inflammatory function within the hematopoietic compartment, in which it restrains production of IL-12 by myeloid cells in response to Helicobacter challenge. A genetic locus controlling colitis susceptibility in mice In addition to the Il10 −/− and TRUC models, we now show that the risk-conferring genotype of Cdcs1 also confers susceptibility to spontaneous colitis in C57BL/6. Was −/− mice (Supplementary Fig. 1a–c ). In both Was −/− and TRUC mice, colitis susceptibility requires homozygosity for the C3H-derived Cdcs1 allele in hematopoietic cells (Supplementary Fig. 1d–e ) [9] . Previously, we mapped the critical region of the Hiccs locus to a 1.71-Mb interval that contains five microRNAs and eight protein-coding genes [3] . We have similarly fine-mapped the susceptibility-controlling region of Cdcs1 in TRUC mice to a congenic interval flanked by the genetic markers D3Mit348 and D3Mit319 (Supplementary Fig. 2 ). This Cdcs1 core region is essentially identical with Hiccs (Fig. 1a ). Therefore, we hypothesized that this locus contains a previously unidentified gene that controls colitis susceptibility in multiple mouse models of IBD. Fig. 1 129.Ra g2 −/− mice rapidly activate interferon-gamma signaling following infection with Hh . a Schematic of the Hiccs locus, which regulates sensitivity to Hh -driven innate colitis. b Colitis phenotypes after Hh infection of B6. Rag1 −/− , 129. Rag2 −/− , or congenic 129. Rag2 −/− mice bearing a Hiccs locus that matches the B6 genotype (129. Hiccs B6 . Rag2 −/− ). c – e Transcriptomic profiling of whole-colon tissue from 129. Rag2 −/− and 129. Hiccs B6 . Rag2 −/− mice 2 days after oral Hh infection ( n = 4 per group). c Tornado plot displaying log 2 fold differences in 129. Rag2 −/− versus 129. Hiccs B6 . Rag2 −/− mice. IFN-γ-regulated genes are indicated in red. d Gene set enrichment analysis (GSEA), showing enrichment of the “interferon-gamma response” hallmark gene set in colon tissue from 129. Rag2 −/− mice. e The top 100 differentially expressed genes (high in 129. Rag2 −/− mice) were analyzed for gene ontology (GO) term enrichment using ClueGO. The most highly enriched GO terms are shown, with lead terms and associated p -values indicated. f RT-qPCR analysis of whole-colon gene expression after Hh infection. Data analyzed by two-way ANOVA ( n = 4 per group per time point). P -values indicate day 2 comparisons corrected with Sidak’s multiple comparisons tests (DF = 17 for each comparison). g IFN-γ secretion by colon explant tissue cultured overnight ex vivo at steady state or following Hh infection. ND no IFN-γ detected in culture supernatant. Data ( Hh day 2) analyzed by Mann–Whitney test ( n = 4 per group/timepoint). Data in c – g are from one experiment Full size image Early IFN-γ response in Hh -treated colitis-susceptible mice A congenic 129SvEv strain carrying the B6 allele of the Hiccs locus (129. Hiccs B6 . Rag2 −/− ) phenocopies the colitis resistance displayed by C57BL/6 mice (Fig. 1b ) [3] . To better understand how the Hiccs locus regulates colitis, we performed transcriptomic analysis of colon tissue from 129. Rag2 −/− and 129. Hiccs B6 . Rag2 −/− mice during the early phase of Hh infection. As early as 2 days post infection, we observed robust induction of inflammatory genes, many of which are known to be interferon-regulated, in 129. Rag2 −/− but not 129. Hiccs B6 . Rag2 −/− mice (Fig. 1c , Supplementary Data 1 ). Indeed, independent gene set enrichment (GSEA) and gene ontology (GO) analyses identified IFN-γ-response genes as being highly enriched in Hh -infected 129. Rag2 −/− mice (Fig. 1d, e ). IFN-γ was highly overexpressed in colon tissue of Hh -infected 129. Rag2 −/− mice at both the mRNA and protein level (Fig. 1f, g ). The genes encoding the p35 and p40 subunits of IL-12 ( Il12a and Il12b ), a critical upstream driver of IFN-γ expression, were similarly overexpressed by 129. Rag2 −/− mice (Fig. 1f ). Alpk1 deficiency confers susceptibility to innate colitis The rapid kinetics of Hh -induced inflammation in 129. Rag2 −/− mice suggest that the Hiccs locus may control some aspect of acute bacterial recognition and effector function. Among Hiccs locus genes, Alpk1 and Tifa have been implicated in bacterial recognition by epithelial cells [12] , [13] , [14] , [15] . Interestingly, while the 129 and B6 alleles of Alpk1 differ by 17 non-synonymous polymorphisms, no such differences exist in Tifa [3] . Therefore, we generated Alpk1 loss-of-function mice on the C57BL/6 background ( Alpk1 −/− ) via CRISPR/Cas9-mediated disruption of Alpk1 exon 10. At steady state, Alpk1 −/− mice were viable, healthy, and showed no obvious immunological phenotypes compared to wild type or heterozygous littermates [16] . Alpk1 −/− mice were then bred with C57BL/6 Rag1 −/− mice to be tested in the Hh -induced innate colitis model (Fig. 2a ). Hh -infected Alpk1 −/− Rag1 −/− animals developed severe inflammation in the caecum and colon, whereas Alpk1 +/− Rag1 −/− mice developed mild inflammation (Fig. 2b, c ), with the largest differences between genotypes occurring in the mid- and distal colon regions (Fig. 2d ). Thus, Alpk1 deficiency causes a colitis-susceptible phenotype similar to that of 129. Rag2 −/− mice, suggesting Alpk1 as a potential regulator of colitis susceptibility in the Hiccs and Cdcs1 loci. Fig. 2 Alpk1-deficient mice are highly susceptible to Hh -induced innate colitis. a Experimental schematic of Hh infection using B6. Rag1 −/− Alpk1 −/− mice or B6. Rag1 −/− Alpk1 +/– littermate controls. b Representative H&E stained mid-colon cross-sections at steady state and after 12 days of Hh infection. Scale bars = 100 μm. c – d Overall colon histopathology scores ( c ) and histopathology scores along the length of the large intestine, from caecum to distal colon ( d ). Steady state ( n = 5), B6. Rag1 −/− Alpk1 −/− + Hh ( n = 5) and B6. Rag1 −/− Alpk1 +/– + Hh ( n = 6). Data shown are from one of three representative experiments and only the Hh -treated groups were analyzed by Mann–Whitney test ( c ) or by two-way ANOVA (genotypes of the Hh infected groups compared, corrected with Sidak’s multiple comparisons test, DF = 52) ( d ). e – f Flow cytometry analysis of cytokine expression by colon lymphocyte and myeloid populations after PMA/ionomycin restimulation. Frequency of IFN-γ expression among ILCs, geometric mean fluorescence intensity (gMFI) of IFN-γ + cells, and frequency of TNF expression among myeloid cells are shown in f . Only the Hh -treated groups were taken into analysis by Mann–Whitney test. g Whole-colon expression of Ifng , IFN-γ-regulated genes, and selected inflammatory cytokines analyzed by RT-qPCR. Only the Hh -treated groups were analyzed by Mann–Whitney test. e – g Data summarize two independent experiments: steady state ( n = 4), B6. Rag1 −/− Alpk1 −/− + Hh ( n = 6) and B6. Rag1 −/− Alpk1 +/– + Hh ( n = 7). h Colon histopathology scores from steady-state mice ( n = 6), Hh -infected B6. Rag1 −/− Alpk1 +/– mice ( n = 15), and B6. Rag1 −/− Alpk1 −/− animals infected with Hh and treated with IgG isotype control antibodies ( n = 12), IL-12p40 neutralizing antibodies ( n = 6), or IL-23R neutralizing antibodies ( n = 6). Data were pooled from two independent experiments and analyzed by two-way ANOVA. P -values indicate treatment comparisons (B6. Rag1 −/− Alpk1 −/− + Hh IgG vs anti-p40 or IgG vs anti-IL23R) corrected with Sidak’s multiple comparisons tests (DF = 159 for each comparison) Full size image In agreement with colon histopathology, total numbers of colonic CD45 + leucocytes, particularly neutrophils, monocytes, and Ly6C + macrophages, were significantly higher in Hh -infected Alpk1 −/− versus Alpk1 +/− animals, as was the frequency of TNFα expression among myeloid cells (Fig. 2e–f , Supplementary Fig. 3a–d ). Our previous study demonstrated that innate lymphoid cells (ILCs) are critical for Hh -induced inflammation in 129. Rag2 −/− mice [3] , [17] . Although, the IFN-γ + ILC frequency in colon tissue from Alpk1 +/− and Alpk1 −/− littermates was similar (Fig. 2e, f ), the intensity of IFN-γ expression in Alpk1 −/− ILCs was significantly increased (Fig. 2e, f ). By contrast, production of IL-22 and IL-17A by colonic Alpk1 −/− ILCs was unaltered or reduced (Supplementary Fig. 3e–g ). Whole-colon tissue of colitic Alpk1 −/− Rag1 −/− mice showed high expression of Ifng , Il12a , Il12b , Il23a , and other inflammatory factors compared to heterozygous littermates (Fig. 2g ). We also observed elevated Il12b mRNA expression in the colons of Hh -infected Alpk1 −/− Rag1 −/− mice using RNAScope in situ hybridization (Supplementary Fig. 3h ) [18] . As with Hh -infected 129. Rag2 −/− mice [19] , [20] , [21] , treatment with an IL-12p40 neutralising antibody, which targets both IL-12 and IL-23, strongly suppressed colonic inflammation in Alpk1 −/− Rag1 −/− mice, while blocking the IL-23 receptor (IL-23R) only partially reduced pathology (Fig. 2h ). Therefore, both IL-12 and IL-23 are non-redundant drivers of Hh -induced colitis in Alpk1 −/− Rag1 −/− mice. The role of Alpk1 in a lymphocyte-replete model of colitis Having found a critical role for Alpk1 in regulating inflammation in a Rag1 -deficient setting, we next assessed its impact on lymphocyte-replete colitis. Hh infection does not induce colitis in wild-type B6 mice unless IL-10 signalling is blocked [22] . We therefore treated Alpk1 +/− and Alpk1 −/− mice with Hh and an IL-10R (IL-10 receptor alpha) blocking antibody to induce colitis (Fig. 3a ). In agreement with results obtained using Rag1 −/− mice, Alpk1 −/− animals developed exacerbated intestinal inflammation based on histological scoring (Fig. 3 b, c), colonoscopy (Fig. 3d ), and total CD45 + lamina propria leucocytes (Fig. 3e ). Interestingly, only complete Alpk1 deficiency resulted in exacerbated pathology, as heterozygous ( Alpk1 +/− ) and wild-type ( Alpk1 +/+ ) littermates displayed comparably modest colitis (Supplementary Fig. 4a ). Consistent with their increased colitis, Alpk1 −/− mice also displayed moderate splenomegaly (Supplementary Fig. 4b ). The increased disease burden in Alpk1 −/− mice was not due to increased intestinal colonization by Hh (Supplementary Fig. 4c ). Fig. 3 Alpk1 deficiency in haematopoietic cells drives exacerbated colitis and intestinal Th1 responses in Hh -infected lymphocyte-replete mice. a Experimental schematic of colitis induced by oral infection with Hh and systemic blockade of the IL-10 receptor (legend applies to b – g ). For panels c , e , and g , data shown summarize two independent experiments: steady state ( n = 9), Hh /αIL-10R-treated Alpk1 +/+ and Alpk1 +/− ( n = 11), and Alpk1 −/− ( n = 6). b Representative H&E stained mid-colon cross-sections at steady state and following 12 days of Hh infection and αIL-10R treatment. Scale bars = 100 μm. c Colon histopathology scores. Only Hh -treated groups analyzed by Mann–Whitney test. d Colonoscopy-based colitis scores from one of two experiments, the Hh -treated groups were analyzed by Mann–Whitney test. Steady state ( n = 6); Hh /αIL-10R-treated Alpk1 +/− ( n = 4); Hh /αIL-10R-treated Alpk1 −/− ( n = 4). e Total live CD45 + colon lamina propria leucocytes in steady state and colitic mice. Hh -treated groups were analyzed by Mann–Whitney test. f – g Flow cytometry analysis of cytokine expression by colon lamina propria CD4 + T cells stimulated with PMA and ionomycin in the presence of brefeldin A. f Representative plots of IFN-γ and IL-17A expression. g Frequencies of IFN-γ + IL-17A − and IFN-γ − IL-17A + cells among total CD4 + T cells, two Hh -treated groups were analyzed by Mann–Whitney test. h – k Analysis of Alpk1 +/− and Alpk1 −/− mice at steady state ( n = 6), or after 2 weeks of treatment with IL-10R neutralizing antibody ( Alpk1 +/− n = 6; Alpk1 −/− n = 4), infection with Hh ( Alpk1 +/− n = 7; Alpk1 −/− n = 6), or treatment with anti-IL-10R antibody and infection with Hh ( Alpk1 +/− n = 4; Alpk1 −/− n = 4). Data represent two independent experiments. Bar charts indicate means ± SEM, compared using multiple t -tests with Holm-Sidak multiple testing correction. h Colonoscopy-based colitis scores. i Whole-colon gene expression analysis by RT-qPCR. j Representative flow cytometry analysis of colonic CD4 + T cells at steady state or after Hh infection without anti-IL-10R treatment. Top panels depict IFN-γ and IL-17A expression after stimulation with PMA/ionomycin and brefeldin-A; bottom panels depict RORγt and FOXP3 expression in unstimulated cells. k Frequencies and absolute numbers of CD4 + IFN-γ + T cells (left two panels). Frequencies of CD4 + FOXP3 + and CD4 + FOXP3 + RORγt + T cells are shown in the right two panels Full size image The Hh + anti-IL10R protocol normally elicits a CD4 + helper T-cell response with mixed Th1 and Th17 characteristics. However, compared to WT or heterozygous controls, intestinal CD4 + T cells of Alpk1 −/− mice were highly skewed towards a Th1 phenotype (IFN-γ + IL-17A – ) following induction of colitis, as measured by cell frequency and IFN-γ expression per cell (Fig. 3 f, g, Supplementary Fig. 4d, e ). In keeping with their similar degree of colitis, wild type and Alpk1 +/− mice showed comparable T cell phenotypes; only Alpk1 −/− mice developed a polarized Th1 response (Supplementary Fig. 4d ). Although IFN-γ was largely co-expressed with TNF-α, frequencies of TNF-α expression were not significantly elevated in Alpk1 −/− T cells (Supplementary Fig. 4f ). In contrast, the frequency of Th17 cells (IFN-γ – IL-17A + ) and their intensity of IL-17A expression was diminished in Alpk1 −/− mice (Fig. 3f, g , Supplementary Fig. 4e ). IL-22 producing CD4 + T cells were also less frequent in Alpk1 −/− mice (Supplementary Fig. 4g ). Boolean gating analysis of cytokine-producing CD4 + T cells confirmed a profound shift in effector phenotype in the absence of Alpk1, with IFN-γ + IL-17A − cells vastly outnumbering other populations (Supplementary Fig. 4h ). Although the total number of colonic FOXP3 + regulatory T cells (Treg) was comparable between Alpk1 −/− and control mice, their frequency among CD4 + T cells was reduced in Alpk1 −/− mice, particularly the FOXP3 + RORγt + subset that is induced in response to Hh (Supplementary Fig. 4i ) [23] . While we observed a similarly Th1-skewed phenotype in the mesenteric lymph nodes of Alpk1 −/− animals, this was not apparent in their peripheral lymph nodes (inguinal/axillary) or spleens (Supplementary Fig. 4j ), suggesting that Alpk1 exerts local control over Th1 immunity. Gene expression analysis of whole-colon tissue confirmed elevated amounts of pro-inflammatory and Th1 cytokines in colitic Alpk1 −/− mice, while expression of Th2 cytokines and IL-10 were reduced relative to WT/heterozygous animals (Supplementary Fig. 4k ). Interestingly, Alpk1 −/− mice displayed a robust intestinal Th1 response and reduced frequency of FOXP3 + RORγt + Treg following Hh infection in the absence of IL-10R blockade (Fig. 3h–k ). This alteration in Th1/Treg balance did not cause marked pathology or recruitment of myeloid leucocytes to the colon, however (Fig. 3h , Supplementary Fig. 4l ). In contrast, Alpk1 −/− mice treated with anti-IL-10R antibody alone did not show any signs of pathology or activation of a Th1 response (Fig. 3h, i, k ). Therefore, Alpk1 deficiency augments the IL-12/Th1 axis and reduces the Treg/Th1 ratio following Hh infection, causing mild immunopathology that is exacerbated in the absence of IL-10 signalling. Alpk1 controls colitis severity via hematopoietic cells Analysis of the Immgen database [24] and FACS-sorted intestinal populations revealed a broad spectrum of Alpk1-expressing cell types, including antigen presenting cells (APCs), epithelial cells, and intestinal stromal cells (Supplementary Fig. 5 ). To determine whether Alpk1 impacts intestinal inflammation via the hematopoietic compartment, we conducted reciprocal bone marrow chimera experiments. Consistent with prior observations of the Hiccs and Cdcs1 loci [3] (Supplementary Fig. 1 - 2 ), irradiated WT mice reconstituted with Alpk1 −/− bone marrow developed more severe Hh + anti-IL-10R-induced colitis in comparison to those that received WT bone marrow (Fig. 4a–c ). Conversely, irradiated WT or Alpk1 −/− animals reconstituted with wild-type bone marrow developed comparable levels of colitis (Fig. 4d–f ), demonstrating that Alpk1 regulates colitis via the hematopoietic compartment. Fig. 4 Control of colitis by Alpk1 depends on its expression in the hematopoietic compartment. a – f Reciprocal bone marrow chimaera experiments in which B6.CD45.1 mice are irradiated and reconstituted with wild type or Alpk1 −/− bone marrow a – c , or wild type and Alpk1 −/− mice are irradiated and reconstituted with wild-type B6.CD45.1 bone marrow d – f . After reconstitution, mice are subjected to Hh + αIL-10R colitis. The Hh -treated groups were compared using Mann–Whitney tests. a – c Colon and caecal histopathology scores ( b ) and frequencies of IFN-γ + IL-17A − and IFN-γ − IL-17A + cells among total colonic CD4 + T cells ( c ). n = 7 recipients of WT bone marrow, n = 6 recipients of Alpk1 −/− bone marrow, and n = 2 steady state. One experiment was performed. d – f Colon and caecal histopathology scores ( e ) and frequencies of IFN-γ + IL-17A − and IFN-γ − IL-17A + cells among total colonic CD4 + T cells ( f ). n = 5 WT recipients, n = 7 Alpk1 −/− recipients, and n = 5 steady state. One experiment was performed Full size image Because CD4 + T-cell responses are largely programmed by APCs, we employed the naive T-cell transfer model of colitis (i.e., adoptive transfer of naive CD4 + T cells to Rag1 −/− hosts) to test whether, in the absence of acute bacterial challenge, deficiency of Alpk1 in APCs could influence the phenotype of expanding T cells. However, transfer of WT T cells to Alpk1 −/− Rag1 −/− or Alpk1 +/− Rag1 −/− hosts resulted in equivalent T-cell differentiation and severity of colitis (Supplementary Fig. 6a–d ). Similarly, no differences were observed between Alpk1 +/+ Rag1 −/− recipients following transfer of Alpk1 −/− or WT T cells (Supplementary Fig. 6e–h ). Thus, Alpk1 deficiency in the absence of a strong microbial driver does not appear to significantly impact CD4 + T-cell differentiation or susceptibility to T-cell-driven colitis. We also tested the role of Alpk1 in another model of colitis that bypasses bacterial stimuli, in which treatment of Rag1 −/− mice with an agonistic anti-CD40 antibody directly activates APCs and induces IL-12/IL-23-mediated pathology [21] . Alpk1 +/− Rag1 −/− and Alpk1 −/− Rag1 −/− mice developed comparable levels of inflammation following anti-CD40 challenge (Supplementary Fig. 6i–n ), providing further evidence that Alpk1 is functionally linked to microbial sensing. Alpk1 regulates Hh -driven IL-12 production by phagocytes Alpk1 has been proposed to affect several distinct cellular pathways [13] , [25] , [26] , [27] , [28] , [29] , yet none explain the pathological effect of its deficiency in the gut. However, our in vivo data suggest that the defect may be related to bacterially induced IL-12 production. Because APCs are the major producers of IL-12, we generated bone marrow-derived macrophages (BMDMs) via culture of bone marrow with GM-CSF (granulocyte-macrophage colony stimulating factor) and examined their response to Hh (Fig. 5a ). After 8 days of culture, flow cytometry analysis revealed no clear differences in differentiation between WT and Alpk1 −/− cells (Supplementary Fig. 7a–c ). Compared to WT cells, Alpk1 −/− BMDMs secreted more IL-12 following exposure to Hh , whereas IL-23 production was similar (Fig. 5b ). At the mRNA level, expression of Il12a and Il12b , but not Il23a , was significantly increased in Alpk1 −/− BMDMs (Fig. 5c ). IL-12 secretion by Hh was blocked in the presence of anti-TLR2 antibody (Fig. 5b ), suggesting that Alpk1 mediates signal transduction downstream of TLR2 and upstream of Il12a / Il12b transcription. Interestingly, pure TLR2 and TLR4 agonists, such as Pam3CSK4 and LPS-induced comparable levels of IL-12 in both wild type and Alpk1 −/− cells (Fig. 5b ). Fig. 5 Alpk1 controls Hh -induced immune gene expression by in vitro differentiated macrophages. a Mouse bone marrow-derived macrophages (BMDMs) were differentiated for 8 days in the presence of GM-CSF for subsequent stimulation with Hh and TLR agonists. b Analysis of IL-12 and IL-23 expression by ELISA. Alpk +/− or Alpk1 −/− BMDMs were stimulated with Hh (0.5 O.D. mL − 1 ), Pam3CSK (100 ng mL − 1 ) or LPS (100 ng mL − 1 ) in the presence or absence of a neutralizing anti-TLR2 (0.3 μg mL − 1 ) antibody. Data shown are from pooled bone marrows ( n = 3) from one of two independent experiments, data from the Hh -treated group were analyzed by two-tailed unpaired t -test ( t = 12.99; df = 4). Bars indicate mean of three replicates ± SEM. c Analysis of gene expression by qRT-PCR of BMDMs stimulated with Hh (0.5 O.D. mL − 1 ) for 3 or 8 h. Data are from pooled bone marrows ( n = 3) from one of three independent experiments. P -values corrected using the Holm-Sidak method are shown. Bars indicate mean of three replicates ± SEM. d Volcano plot depicting global gene expression in Hh -treated Alpk1 +/− vs Alpk1 −/− BMDMs. Differences in gene expression between genotypes are expressed as log2 fold change ( x -axis) with adjusted p -values ( y -axis). e Enriched pathways in Alpk1 −/− cells based on top differentially expressed genes in Hh -treated Alpk1 +/− vs Alpk1 −/− BMDMs. The overrepresentation analysis was carried out using the Reactome pathways [46] and the Panther database [45] . f qRT-PCR validation of top differentially expressed genes revealed by RNA-Seq analysis in Alpk1 +/− and Alpk1 −/− BMDMs. Data shown are from pooled bone marrows ( n = 3) from one of two independent experiments, analysed by unpaired t -test. Bars indicate mean of three replicates ± SEM Full size image Transcriptomic analysis of Alpk1-regulated genes To examine the role of Alpk1 in an unbiased manner, we compared whole transcriptomes of Hh -treated wild type and Alpk1 −/− BMDMs using RNA sequencing. Under resting conditions, the transcriptomes of Alpk1 −/− and Alpk1 +/− cells were almost indistinguishable by tSNE (t-stochastic neighbour embedding) analysis (Supplementary Fig. 8a ), with 32 genes (including Alpk1 itself) showing a statistically significant difference, and only 9 > 2-fold (Supplementary Fig. 8b , Supplementary Data 2 ). This confirms that Alpk1 did not dramatically affect the differentiation of BMDMs in vitro. 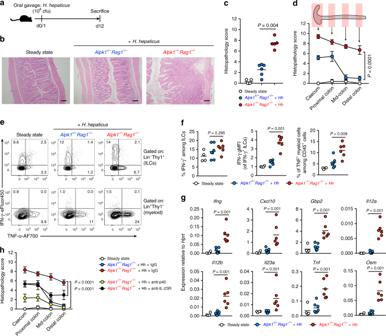Fig. 2 Alpk1-deficient mice are highly susceptible toHh-induced innate colitis.aExperimental schematic ofHhinfection using B6.Rag1−/−Alpk1−/−mice or B6.Rag1−/−Alpk1+/–littermate controls.bRepresentative H&E stained mid-colon cross-sections at steady state and after 12 days ofHhinfection. Scale bars = 100 μm.c–dOverall colon histopathology scores (c) and histopathology scores along the length of the large intestine, from caecum to distal colon (d). Steady state (n= 5), B6.Rag1−/−Alpk1−/−+Hh(n= 5) and B6.Rag1−/−Alpk1+/–+Hh(n= 6). Data shown are from one of three representative experiments and only theHh-treated groups were analyzed by Mann–Whitney test (c) or by two-way ANOVA (genotypes of theHhinfected groups compared, corrected with Sidak’s multiple comparisons test, DF = 52) (d).e–fFlow cytometry analysis of cytokine expression by colon lymphocyte and myeloid populations after PMA/ionomycin restimulation. Frequency of IFN-γ expression among ILCs, geometric mean fluorescence intensity (gMFI) of IFN-γ+cells, and frequency of TNF expression among myeloid cells are shown inf. Only theHh-treated groups were taken into analysis by Mann–Whitney test.gWhole-colon expression ofIfng, IFN-γ-regulated genes, and selected inflammatory cytokines analyzed by RT-qPCR. Only theHh-treated groups were analyzed by Mann–Whitney test.e–gData summarize two independent experiments: steady state (n= 4), B6.Rag1−/−Alpk1−/−+Hh(n= 6) and B6.Rag1−/−Alpk1+/–+Hh(n= 7).hColon histopathology scores from steady-state mice (n= 6),Hh-infected B6.Rag1−/−Alpk1+/–mice (n= 15), and B6.Rag1−/−Alpk1−/−animals infected withHhand treated with IgG isotype control antibodies (n= 12), IL-12p40 neutralizing antibodies (n= 6), or IL-23R neutralizing antibodies (n= 6). Data were pooled from two independent experiments and analyzed by two-way ANOVA.P-values indicate treatment comparisons (B6.Rag1−/−Alpk1−/−+HhIgG vs anti-p40 or IgG vs anti-IL23R) corrected with Sidak’s multiple comparisons tests (DF = 159 for each comparison) In contrast, 599 genes were significantly differentially expressed between the genotypes after Hh stimulation (adjusted p -value <0.05; 67 genes with >2-fold change), including Il12a and Il12b (Fig. 5d , Supplementary Fig. 8b , Supplementary Data 2 ). Pathway enrichment and clustering analyses of the top upregulated genes in Hh -treated Alpk1 −/− cells revealed enrichment of processes related to IL-12 signalling, regulatory interactions between immune cells (e.g., components of CD200R and CD300 signalling pathways), chemokine signalling, and the extracellular matrix (Fig. 5e , Supplementary Fig. 8c , Supplementary Data 2 ). Expression of selected genes at the mRNA level was confirmed using qPCR (Fig. 5f ). Precisely how Hh triggers TLR2 and downstream IL-12 production in mouse BMDMs is unclear. We found that classical TLR and C-type lectin receptor (CLR) agonists, including LPS, CpG, zymozan, and heat-killed mycobacteria, induced comparable IL-12 expression in wild type and Alpk1 −/− BMDMs (Supplementary Fig. 8d ). Assessment of key signalling molecules in the TLR2 pathway, including MAPK kinases and NF-κB revealed no differences between wild type and Alpk1 −/− cells after Hh stimulation (Supplementary Fig. 8e ). Alpk1 expression in human inflammatory bowel disease We previously reported that Alpk1 expression is detectable in murine macrophages under steady-state conditions, but can be further induced by stimulation with LPS or Hh [3] . IFN-γ stimulation similarly increases Alpk1 expression in mouse BMDMs (Supplementary Fig. 8f ). Consistent with these findings, ALPK1 mRNA is highly expressed in the inflamed intestinal mucosa of patients with IBD relative to tissue from healthy control donors in three independent cohorts (Fig. 6a ). Notably, ALPK1 expression in IBD tissue was closely correlated with that of Th1-related cytokines ( IFNG , IL12A , IL12B , and CXCL10 ) but not Th2 or Th17 cytokines ( IL4 , IL13 , and IL17A ) (Fig. 6b ). Thus, in addition to regulation by pattern recognition receptors, Alpk1 expression may be induced by IFN-γ signalling as part of a negative feedback mechanism to limit the intensity of IL-12 production and downstream Th1 immunity. Fig. 6 Alpk1 expression is elevated in inflamed mucosa of IBD patients and correlates with expression of Th1 signature genes. a ALPK1 mRNA expression in intestinal biopsies of healthy controls or IBD patients from three independent publicly available cohorts described in Materials and Methods (Cohort A, GSE4183; Cohort B, GSE16879; Cohort C, GSE57945). Groups were compared by Mann–Whitney test (cohorts A and B) or Kruskal–Wallis test with Dunn’s multiple comparisons tests (cohort C). Bars indicate mean z -scores ± SEM. b RNA-seq gene expression analysis of ileal biopsies from healthy control ( n = 42) and ileal CD patients (Cohort C). CD samples were stratified by relative ALPK1 expression into three equally sized groups ( n = 54 per group) and compared using the Kruskal–Wallis test. Bars indicate mean log 2 RPKM values ± 95% CI, normalized to the control mean Full size image In this study, we have identified Alpk1 as a negative regulator of intestinal inflammation. We demonstrate that Alpk1-deficient mice infected with a pathobiont Helicobacter hepaticus ( Hh ) develop an unusually potent Th1 CD4 + T-cell response and exacerbated colitis in the absence of IL-10 signalling. Unlike IFN-γ-producing Th1 cells, the frequencies of FOXP3 + regulatory and IL-17-producing (Th17) CD4 + T cells are decreased in these animals compared to the wild-type controls. Using bone marrow chimera experiments, we also establish that Alpk1 operates in hematopoietic cells to regulate Hh -induced pathology and the Th1 response. We show that Alpk1 acts as a checkpoint specifically limiting IL-12 production in mononuclear phagocytes, and that this occurs independently of the classical anti-inflammatory cytokine IL-10. Our results suggest distinct immunoregulatory roles for Alpk1 and IL-10 in control of Hh driven inflammation (Fig. 3 ). Although Hh infection of Alpk1 −/− mice resulted in marked skewing of T cell differentiation towards Th1 cells in the colon compared to wild-type mice this was not sufficient to result in severe colitis. By contrast, combined Hh infection and IL-10R blockade caused severe disease with high numbers of colonic Th1 and myeloid cells in Alpk1-deficient mice, as compared to wild-type littermates. These results suggest that Alpk1 and IL-10 represent complimentary checkpoints in the Th1 inflammatory response. Alpk1 may be a critical modulator of CD4 + T cell differentiation through its suppressive effects on IL-12 production, whereas IL-10 is more important for limiting the magnitude of Hh -driven inflammation through controlling the myeloid response [30] . We have shown that Hh stimulation induces elevated IL-12 expression in Alpk1 −/− BMDMs, which is blocked by a neutralising TLR2 antibody (Fig. 5b ). However, stimulation of BMDMs with a TLR2 ligand Pam3CSK4 or other purified pattern recognition receptor ligands induced comparable IL-12 expression in wild type and Alpk1 −/− deficient cells. We speculate that there may be a second, unknown factor under the control of Alpk1 that partners with TLR2 to mediate Hh recognition. Another possibility is that Alpk1 regulates phagocytic clearance of Hh and signalling pathways linked to this process. Interestingly, Alpk1 was initially shown to regulate apical transport in epithelial cells via interaction with myosin Ia [26] . It is possible that a similar machinery is recruited to aid in Hh processing by phagocytes. Deciphering the Alpk1 interactome will be required to investigate this further. Contrary to the data obtained from in vitro cultured human gastric epithelial cells, in which Alpk1 is essential for IL-8 expression induced by certain bacterial pathogens [12] , [13] , we show that Alpk1 deficiency resulted in elevated cytokine expression in BMDMs treated with Hh . This may be explained by a possible cell-type-specific function of Alpk1, as observed for some other inflammatory regulators. For instance, IL-18 signalling in intestinal epithelial cells and lamina propria leucocytes has seemingly opposite effects on intestinal inflammation [31] . Indeed, our bone marrow chimera studies indicate that Alpk1 expression by hematopoietic, but not epithelial cells, is important for control of Hh -induced colitis in vivo (Fig. 4 ). Consistent with this, in vitro analysis showed that Alpk1 can function in macrophages to control Hh -driven IL-12 production. However cell type-specific deletion of Alpk1 will be required to address the context-specific function of Alpk1 in various cell types. Our results identify Alpk1 as the first gene in the Hiccs / Cdcs1 locus with a definitive role in regulating intestinal inflammation. While our data collectively imply that the risk-conferring alleles of Hiccs / Cdcs1 contain a hypomorphic variant of Alpk1 , generation of mice with specific point-mutations in Alpk1 will be required to assess Alpk1 as the causative gene in the Hiccs / Cdcs1 locus. The same genomic interval contains Tifa (TRAF Interacting Protein With Forkhead Associated Domain), which encodes an adaptor protein involved in TNFR/TLR and NLRP3 inflammasome signalling [32] , [33] . We did not focus on Tifa in our studies as there are no non-synonymous nucleotide differences in the Tifa coding region and Tifa mRNA expression levels are similar in myeloid cells between the colitis susceptible and resistant mouse strains [3] . However, TIFA has been recently implicated in sensing of the bacterial metabolite HBP by human epithelial cells, a process that also requires Alpk1 [12] , [13] . Therefore, involvement of TIFA in Alpk1-dependent pathways in the gut cannot be excluded. Considering the distinct roles of Alpk1 in human epithelial and mouse myeloid cells, generation of TIFA knockout mice is essential to explore this axis further. SNPs in the ALPK1 gene have been shown to be associated with inflammatory disease risk in humans [10] , [11] , yet no link has been established between ALPK1 and inflammatory bowel disease. Taking this into account, we examined ALPK1 expression in tissue biopsies from patients with IBD and observed elevated expression compared to healthy individuals. Moreover, Alpk1 expression correlated with the expression of Th1 but not Th2 axis genes in IBD (Fig. 6 ). These data are in line with our findings that Alpk1 expression in BMDMs is induced by both TLR stimulation [3] and IFN-γ, and therefore may represent a negative feedback loop that constrains intestinal Th1 responses. This concept is consistent with the well-known induction of the negative regulator IL-10 by TLR activation, and elevated IL-10 expression found in inflamed tissues. These human findings necessitate additional work to determine the mechanisms that regulate Alpk1 expression, as well as the spatiotemporal pattern of intestinal Alpk1 expression in healthy, inflamed and dysbiotic settings. In summary, we have identified Alpk1 as a critical determinant of murine colitis susceptibility encoded by the Hiccs and Cdcs1 loci. By selectively regulating production of IL-12 downstream of bacterial stimulation, Alpk1 restricts the activation of Th1 immunity in favour of Treg and Th17 responses that maintain homoeostasis. Intriguingly, Alpk1 and IL-10 appear to regulate intestinal homoeostasis via distinct mechanisms, in that Alpk1 controls the nature of intestinal immune responses, while IL-10 controls their magnitude. Thus, loss of Alpk1 function permits aberrant Th1 immunity that, in combination with IL-10 deficiency, causes aggressive and highly destructive colitis (Fig. 7 ). How Alpk1 influences human pathology, and the precise biochemical mechanism by which it regulates expression of inflammatory factors, are key outstanding questions that should be addressed in future studies. Fig. 7 Working model for the role of Alpk1 in controlling gut immune homoeostasis. a TLR2 signaling in response to Helicobacter hepaticus induces expression of Il12a , Il12b , and Il23a in antigen presenting cells (APCs). Alpk1 selectively inhibits expression of Il12a and Il12b , but does not significantly restrain Il23a expression. b In wild-type APCs, control of Il12a and Il12b expression by Alpk1 results in balanced and modest secretion of IL-12p70 and IL-23 in response to H. hepaticus . IL-10 acts independently to further control release of pro-inflammatory cytokines. This results in activation of FOXP3 + RORγt + inducible Tregs and modest induction of Th1 and Th17 effector CD4 + T cells, which does not cause detectable pathology or significant alterations in effector cytokine production in the gut. Additional blockade of IL-10 signaling using an anti-IL10R antibody results in robust activation of a mixed population of Th17 and Th1 effector T cells, recruitment and activation of myeloid cells, and moderate colitis. c In Alpk1-deficient mice, H. hepaticus stimulates potent production of IL-12, which promotes polarized activation of pro-inflammatory Th1 effector T cells at the expense of Tregs and Th17 cells, and mild but detectable inflammation. Following blockade of IL-10R, Th1 cells expand dramatically, inflammatory myeloid populations are recruited to the intestine, and severe colitis ensues. This demonstrates that Alpk1 controls the quality of T cell responses following Helicobacter challenge by restraining IL-12 production and Th1 differentiation, thus promoting a balanced Treg/Th17/Th1 response that maintains homoeostasis. In an Alpk1-deficient setting, Th1 differentiation dominates the Helicobacter -induced T cell response, but IL-10 acts in parallel to restrain Th1 cell expansion and innate inflammation. Removal of both homoeostatic control mechanisms (Alpk1 and IL-10) allows the rapid onset of Th1-driven colitis and ensuing tissue destruction Full size image While this paper was in press, data showing a functional role for Alpk1 in anti-microbial responses were published [34] . CRISPR-assisted generation of ALPK1 knockout mice Using the web based tool [35] four sgRNA, two sgRNA flanking either side of exon 10 of mouse Alpk1 gene (ENSMUSE00001278253) were identified. Deletion of exon 10 generates a frameshift mutation upstream of the alpha-type protein kinase domain. The guide sequences (sgRNAs) were ordered from Sigma Genosys as sense and antisense oligonucleotides and annealed before individually cloning into the T7 expression vector (kind gift from Sebastian Gerety). Following plasmid linearization, RNA was transcribed using a MEGAshortscript T7 Transcription Kit (Thermo Fisher Scientific) and column purified (RNeasy, Qiagen). The humanised Cas9 protein developed by Mali et al. [36] was modified by replacing the CMV promotor with a dual CAG-T7 promotor cassette (kind gift from Katharina Boroviak), thereby allowing expression in the mouse zygote and in vitro transcription of Cas9 mRNA. The vector was linearised and subjected to mMESSAGE mMACHINE® T7 ULTRA Transcription (Thermo Fisher Scientific) before column purification (RNeasy, Qiagen). 75 ngs of Cas9 mRNA, 9.3ngs each of 4 guides was injected into the cytoplasm of fertilised C57BL6n oocytes and transferred into CBAB6F1/J recipients. All applicable European, national, and institutional guidelines for the care and use of animals were followed. All procedures performed in studies involving animals were in accordance with the ethical standards of the Sanger Institute. Mice Wild-type C57BL/6J (referred to elsewhere in the manuscript as B6), 129S6/SvEvTac-Rag2 tm1Fwa and the congenic strain 129.C3BR17.rag [3] (129. Rag2 −/− and 129 .Hiccs B6 . Rag2 −/− , respectively), C57BL/6. Alpk1 em2Wtsi ( Alpk1 −/− ), B6.SJL- Ptprc a Pepc b / BoyJ (B6.CD45.1), C57BL/6. Rag1 −/− (B6. Rag1 −/− ) and C57BL/6. Alpk1 −/− Rag1 −/− (B6. Alpk1 −/− Rag1 −/− ) mice were bred and maintained under specific pathogen free conditions in an accredited animal facility at the University of Oxford and the experiments were conducted in accordance with the UK Scientific Procedures Act of 1986 under a Project License (PPL) authorized by the UK Home Office Animal Procedures Committee. For experiments involving Alpk1 −/− mice, knockout animals and wild type/heterozygous littermate controls were co-housed. 129SvEvS6. Rag2 −/− and R17 congenic strains were bred separately and for experiments the mice from both strains were co-housed after weaning for at least a month before experiments. For genotyping of Alpk1 knockout mice the following primers were used: Alpk1_DF4 GGAGGGGGAGAGAAGTTTGT, Alpk1_DR3 GTCCCTATTCCATCCCTTTTG and Alpk1_ER1 GTCAGGAGGCCAATCTCAAA, with the DF4/ER1 PCR detecting the wild-type Alpk1 allele (190 bp band) and the DF4/DR3 PCR—the Crispr-mutated allele (150 bp band). To ensure maintenance of the Cdcs1 BC-R2 interval during crossing, Was −/− Cdcs1 +/+ mice were genotyped at the D3Mit49 and D3Mit348 loci using the following primers: D3Mit49 - FCTTTTCTCGCCCCACTTTC D3Mit49 - RTCCTTTTAGTTTTTGATCCTCTGG D3Mit348 - FCATCATGCATACTTTTTTCCTCA D3Mit348 - RGCCAAATCATTCACAGCAGA Cg- Tbx21 tm1Glm Rag2 tm1Fwa (T-bet −/− Rag2 −/− , TRUC) mice have been backcrossed to a C57BL/6J (B6) background for at least 10 generations. Congenic TRUC mice carrying the colitogenic Cdcs1 c QTL from C3H/HeJBir mice on a C67BL/6J background [9] were generated by backcrossing BCR3 mice (B6.Cg- Il10 tm1Cgn Cdcs1 ( D3Mit11-D3Mit19 )/JZtm) [6] to the C57BL/6 TRUC line. The TRUC.Cdcs1 c mice initially contained between 8 and more than 26 Mbp of C3H/HeJBir-derived genomic sequence (D3Mit78-D3Mit291) and were further backcrossed to C57BL/6 TRUC mice to generate additional mutants. All mice were housed in microisolator cages in a specific pathogen-free animal facility at the Harvard T.H. Chan School of Public Health. Studies were performed according to institutional and NIH guidelines for humane animal use. Sulfatrim (Sulfamethoxazole 1 g L −1 + Trimethoprim 0.2 g L −1 ; Hitech Pharmacal, Amityville, NY) was added to the drinking water. Mice were genotyped between 2 and 3 weeks, and weaned between 3 and 4 weeks of age. Both male and female mice were used in approximately equal proportions for all experiments. For antibody blockade experiments, mice were randomized to allow for at least two treatments represented in each cage of animals. Minimum sample size of six animals per experimental group (3 for steady state) was determined based on experience with colitis models. Bone marrow chimeras For BM chimera experiments with CD45.1 and Alpk1 knockout mice, recipient mice were lethally irradiated (2 × 550 rads/5.5 Gys) before reconstitution with BM from the indicated donor line. BM was aseptically collected from tibia and femur of the respective donor strain, and 5 × 10 6 cells were injected into the tail vein of the irradiated recipients. Mice were allowed to reconstitute for 8 wk before being infected with H. hepaticus . For TRUC mice, 6–7-week-old recipient mice were lethally irradiated with 800 rad (BALB/c TRUC) or 900 rad (C57BL/6 TRUC). Recipient mice were injected in the lateral tail vein with 2 × 10 6 donor cells in PBS. Mice were killed 20 weeks after BM reconstitution. Chimerism determined by flow cytometric analysis of peripheral blood using H-2K b and H-2K d specific antibodies (Biolegend) was >95% in all animals. BMDM cultures Extracted bone marrow cells were plated at density of 7 × 10 6 cells per 10 cm bacteriological dish and cultured for 7 days in RPMI (Sigma) medium supplemented with Pen-Strep antibiotics (Sigma), 10% FCS (Gibco), 50 μM β-mercaptoethanol (Gibco), GlutaMax TM (Invitrogen) and 20 ng mL − 1 of murine GM-CSF (Peprotech, #315-03). The medium was topped up after 4 days of culture. On day 8, BMDMs were plated in round bottomed 96-well plates at density of 1.5 × 10 5 cells/well and the following day the BMDMs were treated with various microbial stimuli in the presence of 5 ng mL − 1 recombinant mouse IFNγ (Peprotech, #315-05) for 3 h, 8 h, or 24 h. Hh (defrosted bacterial pellets) was used at 0.5 OD/well, ultrapure LPS from E. coli O111:B4 at 10 ng mL − 1 (#tlrl-3pelps), Pam3CSK4 (#tlrl-pms)—100 ng mL − 1 , zymozan (TLR2/dectin-1 agonist, #tlrl-zyn)—1 μg mL − 1 , ODN1826—0.2 μg mL − 1 (CpG, TLR9 agonist, #tlrl-1826), HKMT—10 μg mL − 1 (Mincle agonist, #tlrl-hkmt-1), neutralising anti-mouse TLR2 antibody (clone C9A12, # mabg-mtlr2)—0.3 μg mL − 1 (all from Invivogen). Cytokine expression in the culture supernatant was determined using mouse IL-12 Duoset ELISA kit (RnD Systems) and mouse IL-23 ELISA Ready-SET-Go!™ Kit (eBioscience). Western blot analysis Cell lysates were diluted in the sample buffer (2X, 0.05% bromophenol blue, 20% glycerol, 4% SDS, 0.25 M Tris-HCl, pH 6.8 and 200 mM DTT) and separated by SDS PAGE using precast 4–12% denaturing gels (Invitrogen), immunoblotted and the protein bands were visualized using Amersham ECL detection system (GE Healthcare). Antibodies were from Cell Signalling—pT202/Y204-ERK1/2 (clone D13.14.4E, #4370), pT180/Y182-p38 (clone 3D7, #9215), pT581-MSK1 (#9595), pS473-Akt1 (clone D7F10, #9018), pThr183/Tyr185-JNK (#9251), Sigma—total β-actin (#A1978), Abcam—pS536-RelA (#ab86299). T-cell transfer model of colitis B6. Rag1 −/− mice were injected intraperitoneally (i.p.) with 0.2 × 10 6 FACS-sorted naive CD45RB high CD4 + T cells derived from mouse spleens. Mice were monitored bi-weekly for weight loss. 6–8 weeks after the injections, after the weight loss was approaching 20%, mice were killed and the extent of colitis was analysis by FACS and histology. αCD40 model of murine colitis To induce acute innate colitis, C57BL/6 Rag1 −/− mice were injected intraperitoneally with 50 μg of αCD40 IgG2a mAb (clone FGK45, BioXCell, West Lebanon, NH). Weight loss was monitored daily. Two days post αCD40 injection mice were killed to characterise the extent of colitis. Hh-driven colitis models and in vivo treatments Helicobacter hepaticus, Hh NCI-Frederick isolate 1A (strain 51449) was grown on blood agar plates containing 7% laked horse blood (Thermo Scientific) and trimethoprim, vancomycin and polymixin B (all from Oxoid) under microaerophilic conditions. Cultures were expanded for 3–4 days in TSB (Oxoid) containing 10% FCS (Gibco) and the above antibiotics to OD 0.4–0.5 before collection for oral gavaging. Mice were fed 1 × 10 8 colony forming units (c.f.u.) of H. hepaticus by oral gavage delivered with a 22G curved blunted needle on days 0 and 1 of the experiment (innate model, 129 . Rag2 −/− , 129 HiccsB6 . Rag2 −/− , C57BL/6 Rag1 −/− , and C57BL/6 Alpk1 −/− Rag1 −/− mice). In experiments involving Alpk1 −/− mice on the replete Rag1 +/+ background, 1 mg of an IL‑10R blocking antibody (clone 1B1.2) was administered as an intraperitoneal injection once weekly starting at day 0 of Hh infection. 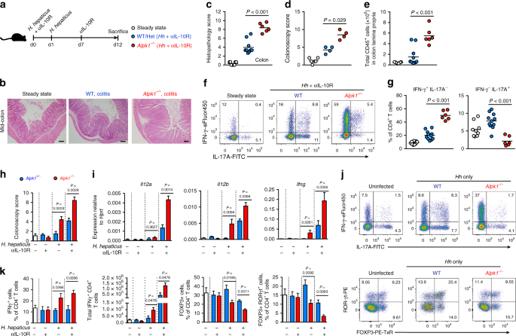Fig. 3 Alpk1 deficiency in haematopoietic cells drives exacerbated colitis and intestinal Th1 responses inHh-infected lymphocyte-replete mice.aExperimental schematic of colitis induced by oral infection withHhand systemic blockade of the IL-10 receptor (legend applies tob–g). For panelsc,e, andg, data shown summarize two independent experiments: steady state (n= 9),Hh/αIL-10R-treatedAlpk1+/+andAlpk1+/−(n= 11), andAlpk1−/−(n= 6).bRepresentative H&E stained mid-colon cross-sections at steady state and following 12 days ofHhinfection and αIL-10R treatment. Scale bars = 100 μm.cColon histopathology scores. OnlyHh-treated groups analyzed by Mann–Whitney test.dColonoscopy-based colitis scores from one of two experiments, theHh-treated groups were analyzed by Mann–Whitney test. Steady state (n= 6);Hh/αIL-10R-treatedAlpk1+/−(n= 4);Hh/αIL-10R-treatedAlpk1−/−(n= 4).eTotal live CD45+colon lamina propria leucocytes in steady state and colitic mice.Hh-treated groups were analyzed by Mann–Whitney test.f–gFlow cytometry analysis of cytokine expression by colon lamina propria CD4+T cells stimulated with PMA and ionomycin in the presence of brefeldin A.fRepresentative plots of IFN-γ and IL-17A expression.gFrequencies of IFN-γ+IL-17A−and IFN-γ−IL-17A+cells among total CD4+T cells, twoHh-treated groups were analyzed by Mann–Whitney test.h–kAnalysis ofAlpk1+/−andAlpk1−/−mice at steady state (n= 6), or after 2 weeks of treatment with IL-10R neutralizing antibody (Alpk1+/−n= 6;Alpk1−/−n= 4), infection withHh(Alpk1+/−n= 7;Alpk1−/−n= 6), or treatment with anti-IL-10R antibody and infection withHh(Alpk1+/−n= 4;Alpk1−/−n= 4). Data represent two independent experiments. Bar charts indicate means ± SEM, compared using multiplet-tests with Holm-Sidak multiple testing correction.hColonoscopy-based colitis scores.iWhole-colon gene expression analysis by RT-qPCR.jRepresentative flow cytometry analysis of colonic CD4+T cells at steady state or afterHhinfection without anti-IL-10R treatment. Top panels depict IFN-γ and IL-17A expression after stimulation with PMA/ionomycin and brefeldin-A; bottom panels depict RORγt and FOXP3 expression in unstimulated cells.kFrequencies and absolute numbers of CD4+IFN-γ+T cells (left two panels). Frequencies of CD4+FOXP3+and CD4+FOXP3+RORγt+T cells are shown in the right two panels For in vivo cytokine blockade experiments, mice were injected intraperitoneally with 0.8 mg IL-23R blocking mAb (D. Cua, Merck, Kenilworth, NJ), or anti-IL-12p40 (clone CB17.8.20) or an isotype control antibody (clone GL117) once weekly starting a day before Hh infection. Scoring of mouse colitis Colonoscopy to assess colitis severity was performed and scored according to the methods of Becker et al. [37] . Histological assessment of colitis severity was performed following the established procedures [38] . Briefly, formalin-fixed paraffin-embedded cross-sections of proximal, middle, and distal colon were stained with haematoxylin and eosin and graded on a scale of 0–3 for four parameters: epithelial hyperplasia and goblet cell depletion, leucocyte infiltration, area affected, and features of severe disease activity. Common severity features include crypt abscess formation, submucosal leucocyte infiltration, and interstitial oedema. Scores for each criterion are added to give an overall score of 0–12 per colon section. Data from the three colon regions are then averaged to give an overall score. Scoring was conducted in a blinded fashion and confirmed by an independent blinded observer. Interobserver Pearson correlation coefficients ranged from 0.8 to 0.9. Photomicrographs of H&E stained colon sections were taken with a Coolscope Slide Scanner (Nikon). For TRUC mice scoring, the histological parameters were mononuclear cell infiltration, polymorphonuclear cell infiltration, epithelial hyperplasia, and epithelial injury were scored as absent (0), mild (1), moderate (2), or severe (3), giving a total score of 0–12 [9] . Mouse colon tissue preparation and cell isolation LPLs were isolated following established procedures [39] . 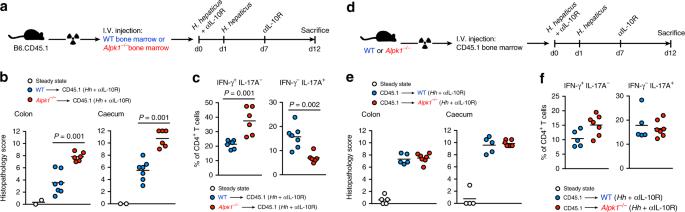Fig. 4 Control of colitis by Alpk1 depends on its expression in the hematopoietic compartment.a–fReciprocal bone marrow chimaera experiments in which B6.CD45.1 mice are irradiated and reconstituted with wild type orAlpk1−/−bone marrowa–c, or wild type andAlpk1−/−mice are irradiated and reconstituted with wild-type B6.CD45.1 bone marrowd–f. After reconstitution, mice are subjected toHh+ αIL-10R colitis. TheHh-treated groups were compared using Mann–Whitney tests.a–cColon and caecal histopathology scores (b) and frequencies of IFN-γ+IL-17A−and IFN-γ−IL-17A+cells among total colonic CD4+T cells (c).n= 7 recipients of WT bone marrow,n= 6 recipients ofAlpk1−/−bone marrow, andn= 2 steady state. One experiment was performed.d–fColon and caecal histopathology scores (e) and frequencies of IFN-γ+IL-17A−and IFN-γ−IL-17A+cells among total colonic CD4+T cells (f).n= 5 WT recipients,n= 7Alpk1−/−recipients, andn= 5 steady state. One experiment was performed Briefly, mouse colons were washed with EDTA to remove epithelium and digested with collagenase VIII to liberate cell populations. Tissue digests were separated by centrifugation on a 40%/80% Percoll (Sigma) gradient. Cells at the 40%/80% interface were collected as the lamina propria leucocyte enriched fraction. Colon explant cultures 3 mm segments isolated from a middle part of mouse colon were cultured overnight in RPMI media supplemented with Pen-strep antibiotics (Sigma), 10% FCS (Gibco) and 50 μM β-mercaptoethanol (Gibco). IFNγ was quantified in the supernatant by enzyme-linked immunosorbent assay (ELISA, R&D Systems, UK) and normalized to explant weight (mg of tissue). Quantitation of H. hepaticus using real-time PCR DNA was purified from caecal contents taken from H. hepaticus –infected mice using the DNA Stool kit (Qiagen). H. hepaticus DNA was determined using a Q-PCR method based on the cdtB gene [40] . RNA extraction, cDNA synthesis, and qPCR Tissues were disrupted using lysis beads and a homogenizer unit (Precellys, UK) in the RLT buffer (Qiagen, UK). Sorted or cultured cells were lysed directly in the RLT buffer and homogenized by pipetting. RNA was isolated using RNEasy Mini or Micro kits (Qiagen, UK) followed by reverse transcription using random primers (Applied Biosystems, UK). Quantitative PCR (qPCR) was performed using Taqman assays (Applied Biosystems) and PrecisionPlus Mastermix (Primer Design, UK) on a ViiA7 384-well real-time PCR detection system (Applied Biosystems). All expression levels were normalized to an internal house-keeping gene Hprt and calculated as 2 (CT Hprt −CTgene) . Microarray analysis Expression profiles of colon tissues from 129. Rag2 −/− and 129. HiccsB6 . Rag2 −/− were obtained using Illumina MouseWG-6-V2 microarrays ( n = 4 for each condition). Array signal intensities were background adjusted, transformed using the variance-stabilizing transformation and quantile normalized using Lumi [41] from R/Bioconductor. Probes were retained if they were expressed significantly above background levels in at least four samples. This resulted in the analysis of 20,997 probes representing 15,443 genes. Differential expression analysis was performed using the empirical Bayes method in LIMMA [42] . Significance was defined as a Benjamini-Hochberg adjusted P -value <0.05. RNA sequencing analysis PolyA-selected RNA from in vitro differentiated macrophages (Fig. 5 ) from pooled bone marrows from three mice (split into three technical replicates per condition) was used to prepare cDNA libraries (in-house dUTP protocol) that were subject to next-generation sequencing (Illumina HiSeq4000; 75 bp; minimum of 50M read pairs per sample). Mapping was performed using HISAT2 [43] (two pass strategy to incorporate novel splice-sites) together with an index built from the mouse genome (mm10) and Ensembl transcript annotations (version 88). Differential expression analysis was performed using read counts (quantitated with featureCounts [44] ) and the DESeq2 algorithm [45] (local fit). P -values were adjusted for multiple-testing using the Benjamini-Hochberg correction. Pathways and gene set enrichment analysis We tested for the enrichment of pathways that were differentially upregulated at day 2 of Hh infection in 129. Rag2 −/− and 129 HiccsB6 . Rag2 −/− mice. Gene set enrichment analysis (GSEA) was conducted using the GSEA desktop program; Hallmark gene sets were downloaded from the Molecular Signatures Database ( http://software.broadinstitute.org/gsea/msigdb/collections.jsp ). For gene ontology enrichment analysis (focusing on GO_ImmuneSystemProcess and REACTOME terms), the top 100 most significantly differentially expressed genes in 129. Rag2 −/− vs 129 HiccsB6 . Rag2 −/− mice after 2 days of Hh stim were analysed using ClueGO v2.1.7 with a minimum kappa score threshold of 0.5 and right-sided hypergeometric test with Bonferroni step-down correction to identify significant terms. For RNA-Seq, top significant (adj. p -value <0.01) genes differentially expressed in Alpk1 +/− and Alpk1 −/− BMDMs were analyzed using the online tool Panther [46] and Reactome pathways [47] as a source of terms for pathway enrichment analysis. Flow cytometry and cell sorting Mouse cells were stained with combinations of the following monoclonal antibodies, with dilutions/catalogue numbers indicated in brackets, according to manufacturer protocols: B220-PerCP (1/400; RA33-6B2), CCR7-PE (1/100; 4B12), CD4-BV605 (1/200; RM4-5), CD11b-PerCP-Cy5.5 (1/400; M1/70), CD11b-BV510 (1/300; M1/70), CD11c-efluor450 (1/200; N418), CD11c-BV605 (1/200; N418), CD11c-PerCP-Cy5.5 (1/400; N418), CD19-biotin (1/300; 6D5), CD25-PE-Cy7 (1/200; PC61.5), CD40-APC (1/150; 1C10), CD44-BV510 (1/150; IM7), CD45-BV650 (1/400; 30-F11), CD45-BV510 (1/400; 30-F11), CD45-AF700 (1/300; 30-F11), CD45.1-PE-Cy7 (1/200; A20), CD45.2-AF700(1/400; 104), CD45RB-APC (1/150; C363.16A), CD62L-PE (1/150; MEL-14), CD86-FITC (1/150; GL1), CD115-PE-Cy7 (1/100; AFS98), CD117-AF700 (1/150; ACK2), CD135-biotin (1/150; A2F10), F4/80-BV421 (1/150; BM8), FOXP3-PE-TxR (1/150; FJK-16s), Gr1-FITC (1/400; RB6-8C5), IFNγ-ef450 (1/500; XMG1.2), TNF-PE-Cy7 (1/200; MP6-XT22), TNF-AF700 (MP6-XT22), IL-17A-FITC (1/150; TC11-18H10.1), IL-17A-BV605 (1/150; TC11-18H10.1), IL-22-PE (1/150; 1H8PWSR), Ly6C-PE-Cy7 (1/300; HK1.4), MHCII-AF700 (1/200; M5/114.15.2), MHCII-BV785 (M5/114.15.2), RORγT-PE (1/400; Q31-378), Siglec-F-PE (1/200; E50-2440), streptavidin-PE-CF594 (1/500; SP34-2), Thy1.2-PE-Cy7 (1/800; 53-2.1) and TCRβ-BV510 (1/100; H57-597). All antibodies were from eBioscience (UK), Biolegend (UK), Becton Dickinson (UK), or R&D Systems (UK). Dead cells were excluded using efluor-780 fixable viability dye (eBioscience). Samples were acquired on FACS LSR Fortessa and FACS LSRII flow cytometers (Becton Dickinson). Cell sorting was performed using a FACS ARIA III (Becton Dickinson). Data were analyzed using FlowJo (Tree Star, USA). For intracellular cytokine staining, cells were restimulated with PMA (10 ng mL − 1 ; Sigma-Aldrich), ionomycin (1 μg mL − 1 ; Sigma-Aldrich), and 5 µg mL − 1 brefeldin A (Sigma-Aldrich). After 3 h, cells were stained with fixable viability dye and surface markers, fixed with BD FACS Lysing Solution (Becton Dickinson, UK), and stained for intracellular cytokines in permeabilization buffer containing 0.05% saponin (Sigma-Aldrich). For staining FOXP3, cells were stained with fixable viability dye and surface markers prior to fixation and permeabilization using the FOXP3 staining buffer kit (eBioscience) according to manufacturer instructions. Gating strategy employed in the study is shown on Supplementary Fig. 9 . Boolean analysis of cytokine expression by CD4 + T cells was performed using SPICE with default parameters [48] . RNAScope Alpk1 +/− Rag1 −/− and Alpk1 −/− Rag1 −/− mice were untreated ( n = 4) or infected with Helicobacter hepaticus by oral gavage with 1 × 10 8 CFU ( n = 5) and killed after 2 days. Formalin-fixed paraffin-embedded tissues from proximal colons were sectioned at 5 μm and collected onto Superfrost glass slides. Tissue sections were dewaxed in xylene and rehydrated through graded alcohol to water. Antigens were retrieved by boiling the tissue sections in target-retrieval buffer provided by ACD, following the manufacturer’s instructions. For detection of mouse Il12b and Alpk1 mRNA, the RNAScope Multiplex Fluorescent Reagent kit v2 (ACD Europe SRL) was used. For Alpk1 mRNA detection, the probe Alpk1 was custom made to span all exons with the exception of exon 10, which is excised in Alpk1 KO animals. Briefly, paraffin sections were freshly cut, dried for 1 h at 60 °C and dewaxed before mild unmasking with Target Retrieval buffer and protease, as per the manufacturer’s instructions. Pretreated sections were hybridized with specific probes to Il12b and Alpk1 , as well as Ppib and Polr2a (positive control) and irrelevant probe to dapb as a negative control. After hybridization signal amplification, TSA Plus fluorophores (PerkinElmer) were reconstituted and used to develop individual channel signal ( Il12b in C3, Alpk1 in C5). Nuclei were stained with DAPI and sections were cover-slipped with Prolong Gold Antifade mounting medium (Thermo Fisher). Images were acquired using the A1 Zeiss Axioscope (Carl Zeiss™) at ×40 and ×100 magnifications. For final presentation, images were enhanced using Adobe Photoshop to increase contrast between the red ( Alpk1 ) and yellow ( Il12b ) signals to background DAPI signal. All evaluations were performed in a blinded manner. For Il12b mRNA quantification, ×100 magnification images were used to count Il12b (yellow) dots in Alpk1 -expressing cells (red dots). A minimum of 10 individual cells per mouse and per condition was used for quantification. The total number of cells expressing Il12b and Alpk1 in proximal colon was computed using ×40 magnification images. Analysis of patient cohorts Publicly available whole-transcriptome data from intestinal biopsies of healthy controls and patients with IBD were downloaded from the Gene Expression Omnibus web portal. 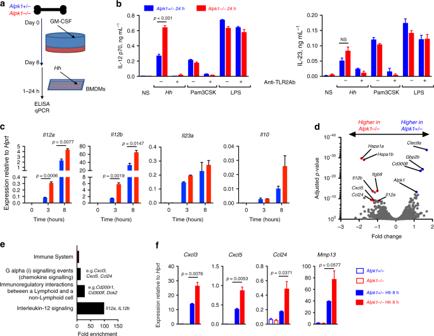Fig. 5 Alpk1 controlsHh-induced immune gene expression by in vitro differentiated macrophages.aMouse bone marrow-derived macrophages (BMDMs) were differentiated for 8 days in the presence of GM-CSF for subsequent stimulation withHhand TLR agonists.bAnalysis of IL-12 and IL-23 expression by ELISA.Alpk+/−orAlpk1−/−BMDMs were stimulated withHh(0.5 O.D. mL−1), Pam3CSK (100 ng mL−1) or LPS (100 ng mL−1) in the presence or absence of a neutralizing anti-TLR2 (0.3 μg mL−1) antibody. Data shown are from pooled bone marrows (n= 3) from one of two independent experiments, data from theHh-treated group were analyzed by two-tailed unpairedt-test (t= 12.99; df = 4). Bars indicate mean of three replicates ± SEM.cAnalysis of gene expression by qRT-PCR of BMDMs stimulated withHh(0.5 O.D. mL−1) for 3 or 8 h. Data are from pooled bone marrows (n= 3) from one of three independent experiments.P-values corrected using the Holm-Sidak method are shown. Bars indicate mean of three replicates ± SEM.dVolcano plot depicting global gene expression inHh-treatedAlpk1+/−vsAlpk1−/−BMDMs. Differences in gene expression between genotypes are expressed as log2 fold change (x-axis) with adjustedp-values (y-axis).eEnriched pathways inAlpk1−/−cells based on top differentially expressed genes inHh-treatedAlpk1+/−vsAlpk1−/−BMDMs. The overrepresentation analysis was carried out using the Reactome pathways46and the Panther database45.fqRT-PCR validation of top differentially expressed genes revealed by RNA-Seq analysis inAlpk1+/−andAlpk1−/−BMDMs. Data shown are from pooled bone marrows (n= 3) from one of two independent experiments, analysed by unpairedt-test. Bars indicate mean of three replicates ± SEM The following datasets were analysed: GSE4183 [49] (cohort A; n = 8 control vs n = 15 IBD; assessed by Mann–Whitney test), GSE16879 [50] (cohort B; n = 12 control vs n = 61 IBD; assessed by Mann–Whitney test), and GSE57945 [51] (cohort C; assessed by Kruskal–Wallis with Dunn’s multiple comparisons test). Statistical analysis Unless otherwise indicated, all bar charts represent means ± S.E.M. Statistical tests were two-sided and specified in figure legends. Differences were considered to be significant when p < 0.05. The non-parametric Mann–Whitney test was used for comparing pathology scores, FACS, ELISA, and Q-PCR data in Hh -treated groups of mice. 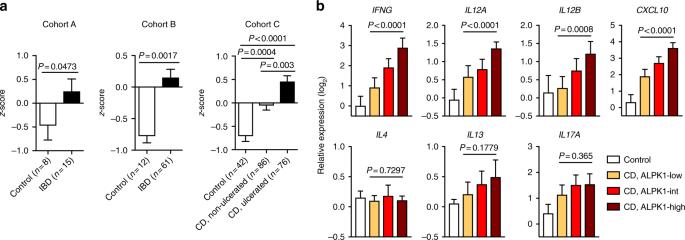Fig. 6 Alpk1 expression is elevated in inflamed mucosa of IBD patients and correlates with expression of Th1 signature genes.aALPK1mRNA expression in intestinal biopsies of healthy controls or IBD patients from three independent publicly available cohorts described in Materials and Methods (Cohort A, GSE4183; Cohort B, GSE16879; Cohort C, GSE57945). Groups were compared by Mann–Whitney test (cohorts A and B) or Kruskal–Wallis test with Dunn’s multiple comparisons tests (cohort C). Bars indicate meanz-scores ± SEM.bRNA-seq gene expression analysis of ileal biopsies from healthy control (n= 42) and ileal CD patients (Cohort C). CD samples were stratified by relativeALPK1expression into three equally sized groups (n= 54 per group) and compared using the Kruskal–Wallis test. Bars indicate mean log2RPKM values ± 95% CI, normalized to the control mean 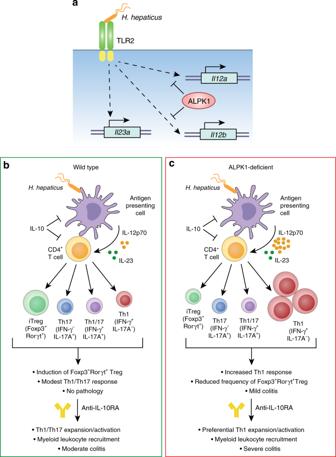Fig. 7 Working model for the role of Alpk1 in controlling gut immune homoeostasis.aTLR2 signaling in response toHelicobacterhepaticusinduces expression ofIl12a,Il12b, andIl23ain antigen presenting cells (APCs). Alpk1 selectively inhibits expression ofIl12aandIl12b, but does not significantly restrainIl23aexpression.bIn wild-type APCs, control ofIl12aandIl12bexpression by Alpk1 results in balanced and modest secretion of IL-12p70 and IL-23 in response toH. hepaticus. IL-10 acts independently to further control release of pro-inflammatory cytokines. This results in activation of FOXP3+RORγt+inducible Tregs and modest induction of Th1 and Th17 effector CD4+T cells, which does not cause detectable pathology or significant alterations in effector cytokine production in the gut. Additional blockade of IL-10 signaling using an anti-IL10R antibody results in robust activation of a mixed population of Th17 and Th1 effector T cells, recruitment and activation of myeloid cells, and moderate colitis.cIn Alpk1-deficient mice,H. hepaticusstimulates potent production of IL-12, which promotes polarized activation of pro-inflammatory Th1 effector T cells at the expense of Tregs and Th17 cells, and mild but detectable inflammation. Following blockade of IL-10R, Th1 cells expand dramatically, inflammatory myeloid populations are recruited to the intestine, and severe colitis ensues. This demonstrates that Alpk1 controls the quality of T cell responses followingHelicobacterchallenge by restraining IL-12 production and Th1 differentiation, thus promoting a balanced Treg/Th17/Th1 response that maintains homoeostasis. In an Alpk1-deficient setting, Th1 differentiation dominates theHelicobacter-induced T cell response, but IL-10 acts in parallel to restrain Th1 cell expansion and innate inflammation. Removal of both homoeostatic control mechanisms (Alpk1 and IL-10) allows the rapid onset of Th1-driven colitis and ensuing tissue destruction Histopathology scores along the length of the large intestine were compared using two-way ANOVA using the Prism software (Graphpad). Where possible, the groups being compared are indicated by a connecting line in figures.